Natural variation ofDt2determines branching in soybean Shoot branching is fundamentally important in determining soybean yield. Here, through genome-wide association study, we identify one predominant association locus on chromosome 18 that confers soybean branch number in the natural population. Further analyses determine that Dt2 is the corresponding gene and the natural variations in Dt2 result in significant differential transcriptional levels between the two major haplotypes. Functional characterization reveals that Dt2 interacts with GmAgl22 and GmSoc1a to physically bind to the promoters of GmAp1a and GmAp1d and to activate their transcription. Population genetic investigation show that the genetic differentiation of Dt2 display significant geographic structure. Our study provides a predominant gene for soybean branch number and may facilitate the breeding of high-yield soybean varieties. Shoot branching is fundamentally important to the growth and productivity of crops [1] . By unconscious or conscious selection of the superior alleles of key genes that confer branching architecture, humans have significantly increased crop yields. One typical example is the selection and utilization of the TEOSINTE BRANCHED1 ( TB1 ) gene during the domestication of maize [2] . TB1 and its orthologs play profound roles in modulating branching architecture via determination of the bud activation potential in plants [1] , [3] , [4] , [5] . Cultivated maize ( Zea mays ) was domesticated from teosinte ( Z. mays ssp. parviglumis ). Largely benefitting from the selection of a higher-expression allele of TB1 , cultivated maize was successfully domesticated as a high-yield crop with a single culm, in contrast to its highly branched ancestor teosinte [6] . Another promising advance is the application of IPA1 in rice. A point mutation in IPA1 leads to an ideal rice plant with fewer tillers, increased plant height, lodging resistance, and thus enhanced grain yield [7] , [8] , [9] . By introducing beneficial ipa1 alleles into widely cultivated cultivars, a series of new elite varieties with higher yields were developed [7] . An increasing number of regulatory genes that control shoot branching are being identified [1] , [10] , providing genetic resources for breeding high-yield crops via molecular design. Soybean ( Glycine max (L.) Merr.) is one of the most important crops that supplies more than half of global oilseed production and approximately one quarter of the world’s plant protein [11] . With the increasing population and continuous improvement in people’s living standards, it was estimated that the soybean yield has to be doubled by 2050 to meet the consumption demands [12] . In contrast to the dramatic increase in yield of major crops, such as rice and wheat, which greatly benefitted from the Green Revolution, soybean yield has not been improved significantly in the past six decades. Modulating branch number, one of the most profound traits that determines the final yield of soybean, is crucial for high-yield soybean breeding [13] . However, to date, the genes associated with soybean branching have seldom been reported [14] . Here, we show that natural variation in Dt2 predominantly determine soybean branching. We also reveal that Dt2 interact with GmAgl22 and GmSoc1a to bind to the promoters of GmAp1a and GmAp1d to regulate their transcriptions. Interestingly, the selection of Dt2 is associated with geographic differentiation. Modulating Dt2 lines resulted in significantly increase of soybean adaptation and yield, which is also associated with its effect on maturity. Natural variation in Dt2 predominantly determines soybean branching To identify the key genes that control branch number in soybean, we phenotyped 2409 accessions from our previous resequencing panel [15] in 2017 and 2018. Phylogenetic and principal-component analysis of the landraces and cultivars did not show significant genetic differentiation (Supplementary Fig. 1a, b ). Genome-wide association study (GWAS) performed using a mixed linear model revealed a stable association signal across the 2 years in a 40 kb interval block on chromosome 18 (Fig. 1a–d and Supplementary Fig. 1d–g ). Within this 40 kb interval, a total of 5 protein-coding genes were annotated according to the reference genome ZH13 [16] , [17] (Fig. 1d ), among which SoyZH13_18g242900 showed higher specific expression at the shoot apical meristem (Supplementary Fig. 2a ), a tissue closely related to the final branching architecture [1] . Therefore, SoyZH13_18g242900 was considered to be the candidate gene controlling branch number in soybean. Fig. 1: GWAS of branch number and haplotype analysis of Dt2 in soybean. a Manhattan plot of GWAS for branch number using 2 years of Blup data of the 2409 accessions. P values are calculated based on linear mixed model in GWAS and the dashed horizontal line indicates the genome-wide significance threshold ( P = 1 × 10 −7.9 ), which is determined by the Bonferroni test. −log 10 P values are plotted against the position of SNPs on 20 chromosomes. b Quantile-quantile plot for the branch number. For quantile-quantile plot, −log 10 -transformed observed P values are plotted against −log 10 -transformed expected P values. c Genome-wide Manhattan plot in the 57–60 Mb region on chromosome 18. The red lead SNPs are shown above the threshold signals. d Linkage disequilibrium plot for SNPs in the 57.80–57.84 Mb region from a continuous association block. Navy blue box, genes. Pink box, candidate gene Dt2 . Asterisk, position of the peak SNP. The color key (white to red) represents linkage disequilibrium value ( r 2 ) accessions. e Gene structure of Dt2 . Two SNPs (−3259th T > C, −2580th T > A) in the promoter and a nonsynonymous SNP (+98th G > A) in the first exon are labeled on the gene sketch. f Haplotype analysis of Dt2 HapI-1 ( n = 1052 accessions), Dt2 HapI-2 ( n = 262 accessions) and Dt2 HapII ( n = 179 accessions). In each box plot (drawn by R 4.1.1 software), the center line indicates the median, the edges of the box represent the first and third quartiles, and the whiskers extend to span a 1.5 interquartile range from the edges. Different letters indicate statistically significant differences at P < 0.05 by one-way ANOVA test. g Promoter activity analysis of Dt2 HapI and Dt2 HapII using sequences 3,400-bp upstream from the translation initiation site ( n = 5 biologically independent replicates), ** P < 0.01, two-sided t -test, and P = 6.0 × 10 −3 . Data in ( f , g ) are the mean ± SEM. Source data are provided as a Source Data file . Full size image SoyZH13_18g242900 , also known as Dt2 , has been found to play important roles in regulating multiple agronomic traits, including stem growth habit, plant height, and flowering time [18] , [19] , [20] . Whether it could modulate branch number has not been investigated. Phylogenetic analysis found that Dt2 belongs to MADS-box transcription factor family and shares high homology with AGL79 in Arabidopsis , a member of the AP1/FUL subfamily (Supplementary Fig. 2c ). Of the association polymorphisms with minor allele frequency (MAF) >0.05, two SNPs from the promoter regions (3259 bp and 2580 bp upstream of the translation start site, respectively) and six SNPs from the introns showed higher association values than the threshold, and a G/A SNP from the first exon that changed amino acid serine to asparagine showed a lower association value than the threshold (Supplementary Fig. 2b ). Based on these higher-value association SNPs and the G/A nonsynonymous SNP, three major haplotypes of Dt2 : Dt2 HapI-1 , Dt2 HapI-2 , and Dt2 HapII were classified in the natural population (Fig. 1e, f ). We found that the accessions harboring Dt2 HapI-1 and Dt2 HapI-2 did not exhibit a significant difference in branch number, whereas Dt2 HapII showed a significantly lower branch number than Dt2 HapI-1 and Dt2 HapI-2 (Fig. 1f ). Transient transcription activity assays suggested that the promoter sequence of Dt2 HapII had significantly higher transcriptional activity than that of Dt2 HapI (Fig. 1g ). We then randomly selected 20 representative natural accessions and investigated the gene expression level of Dt2 and branch number. A negative correlation between the Dt2 expression level and branch number was observed (Supplementary Fig. 3a ). Investigation of a pair of Dt2 near-isogenic lines (NILs) also revealed that the Dt2 HapII line exhibited a significantly decreased branch number than the Dt2 HapI-1 line (Supplementary Fig. 3b, c ). Consistently, quantitative real-time PCR (RT-qPCR) assays showed that Dt2 expression in the Dt2 HapII line was significantly higher than that in Dt2 HapI-1 (Supplementary Fig. 3d ). The above results suggested that the variation at the promoter of Dt2 played an important role in determining branch number in soybean. Functional validation of the role of Dt2 in controlling branch number To validate the function of Dt2 in determining branch number, we knocked out Dt2 in Dong Nong 50 (DN50), a variety harboring Dt2 HapII with a mean of four branches, by the CRISPR/Cas9 system and obtained two independent homozygous knockout lines (named Dt2 CR-1 and Dt2 CR-2 , respectively) (Supplementary Fig. 4 ). Field characterization demonstrated that the Dt2 CR lines exhibited increased branch number compared with the wild type DN50 (Fig. 2a, b, f ). The Dt2 CR lines also showed significantly delayed flowering and maturity, and increased plant height and stem node number, which were consistent with its reported functions [18] , [19] (Fig. 2g and Supplementary Fig. 5a–c ). Moreover, we found that the Dt2 CR lines exhibited multiple yield related trait changes, including higher 100 seed weight, longer seed length and width, and higher grain weight per plant, resulting in significantly increased yield per plot (Fig. 2h and Supplementary Fig. 6a, c–f ). Fig. 2: Dt2 negatively regulates the branch number. a Architecture of DN50 and Dt2 CR plants at the harvest stage. b Branching ability of DN50 and Dt2 CR after harvest. c Architecture of DN50 and Dt2 OE plants at the harvest stage. d Branching ability of DN50 and Dt2 OE after harvest. e Relative expression level of Dt2 in DN50 and different transgenic lines ( n = 3 biologically independent replicates). f Branch number of DN50, Dt2 CR and Dt2 OE lines ( n = 70 biologically independent plants). g Flowering time of DN50, Dt2 CR and Dt2 OE lines ( n = 30 biologically independent plants). DAE indicates days after emergence. h Plot yield of DN50, Dt2 CR and Dt2 OE ( n = 4 biologically independent replicates). The plot area is 10 m 2 . Scale bars in the ( a–d ) are 10 cm. Data in ( e – h ) are the mean ± SEM. Statistical significance is determined using a two-sided t -test. Source data are provided as a Source Data file . Full size image We further overexpressed the coding sequence (CDS) of Dt2 driven by the 35 S promoter in DN50 and obtained two independent transgenic overexpression lines (named Dt2 OE-1 and Dt2 OE-2 , respectively). RT-qPCR assays showed that the expression of Dt2 was increased approximately threefold in the Dt2 OE lines compared to the wild type DN50 (Fig. 2e ). In contrast to the results from the Dt2 CR lines, the Dt2 OE lines exhibited decreased branch number, promoted flowering time (Fig. 2c, d, f, h ) and maturity, decreased plant height, decreased stem node number (Supplementary Fig. 5 ), decreased pod number per plant, and decreased seed length and width, thus exhibiting decreased yield per plot (Fig. 2h and Supplementary Fig. 6b, c–f ). These experiments showed that Dt2 negatively regulated branch number in soybean. Growth state statistics of axillary buds in leaf axils between DN50 and Dt2 CR lines showed that the effect of Dt2 on branch development may be related to inflorescence determinacy (Supplementary Fig. 7 ). Dt2 interacts with GmAgl22 and GmSoc1a Transcriptional profiling of different tissues showed that Dt2 was highly expressed in the lateral buds and shoot tip (Supplementary Fig. 8a ). An in situ hybridization assay demonstrated that Dt2 was specifically expressed in the axillary meristem and shoot apical meristem (Supplementary Fig. 8b ). 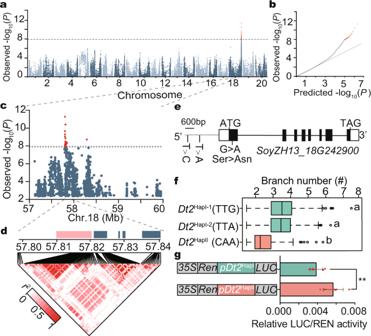Fig. 1: GWAS of branch number and haplotype analysis of Dt2 in soybean. aManhattan plot of GWAS for branch number using 2 years of Blup data of the 2409 accessions.Pvalues are calculated based on linear mixed model in GWAS and the dashed horizontal line indicates the genome-wide significance threshold (P= 1 × 10−7.9), which is determined by the Bonferroni test. −log10Pvalues are plotted against the position of SNPs on 20 chromosomes.bQuantile-quantile plot for the branch number. For quantile-quantile plot, −log10-transformed observedPvalues are plotted against −log10-transformed expectedPvalues.cGenome-wide Manhattan plot in the 57–60 Mb region on chromosome 18. The red lead SNPs are shown above the threshold signals.dLinkage disequilibrium plot for SNPs in the 57.80–57.84 Mb region from a continuous association block. Navy blue box, genes. Pink box, candidate geneDt2. Asterisk, position of the peak SNP. The color key (white to red) represents linkage disequilibrium value (r2) accessions.eGene structure ofDt2. Two SNPs (−3259th T > C, −2580th T > A) in the promoter and a nonsynonymous SNP (+98th G > A) in the first exon are labeled on the gene sketch.fHaplotype analysis ofDt2HapI-1(n= 1052 accessions),Dt2HapI-2(n= 262 accessions) andDt2HapII(n= 179 accessions). In each box plot (drawn by R 4.1.1 software), the center line indicates the median, the edges of the box represent the first and third quartiles, and the whiskers extend to span a 1.5 interquartile range from the edges. Different letters indicate statistically significant differences atP< 0.05 by one-way ANOVA test.gPromoter activity analysis ofDt2HapIandDt2HapIIusing sequences 3,400-bp upstream from the translation initiation site (n= 5 biologically independent replicates), **P< 0.01, two-sidedt-test, andP= 6.0 × 10−3. Data in (f,g) are the mean ± SEM. Source data are provided as aSource Data file. To identify the protein interaction partners of Dt2, we carried out a yeast two-hybrid (Y2H) assay by screening the cDNA library constructed from the lateral buds and identified 136 unique cDNA clones that corresponded to 28 genes (Supplementary Table 1 ). Of the interacting proteins, an ortholog of Arabidopsis SHORT VEGETATIVE PHASE (SVP)/AGL22, named GmAgl22 in this study, showed more repeats and was of interest to us. GmAgl22 encodes a MADS-box transcription factor in Arabidopsis and functions as a floral repressor in the thermosensory pathway [21] , [22] , [23] . The interaction between Dt2 and GmAgl22 was further confirmed by point-to-point Y2H, bimolecular florescence complementation (BiFC), split luciferase complementation (split-LUC) and coimmunoprecipitation (Co-IP) assays (Fig. 3a–c and Supplementary Fig. 9a, b ). Detailed investigation demonstrated that the K-box domain of Dt2 was essential for the physical interaction between Dt2 and GmAgl22 (Supplementary Fig. 9d ). In addition, we found that GmAgl22 could interact with itself in Y2H, split-LUC and Co-IP assays (Supplementary Fig. 10a–c ), indicating that the protein develops dimers or polymers to exert its function. A previous study reported that Dt2 could interact with GmSoc1a to affect the soybean growth habit [18] , [24] . We suspected that GmAgl22 could also interact with GmSoc1a, which was then confirmed by Y2H, BiFC, split-LUC and Co-IP assays (Fig. 3d–f and Supplementary Fig. 9c ). Expression pattern analysis found that GmAgl22 and GmSoc1a were highly expressed in the lateral bud and shoot tips (Supplementary Fig. 10d, e ). In situ hybridization assays demonstrated that GmAgl22 and GmSoc1a , similar to Dt2 , were specifically expressed in the axillary meristem in different developmental stages (Supplementary Fig. 11 ). Fig. 3: Dt2, GmAgl22 and GmSoc1a could interact with each other and affect the branch number. a Interaction between Dt2 and GmAgl22 in the yeast two-hybrid assay. Transformed yeast cells are grown on DDO (Trp/Leu) or QDO (Trp/Leu/His/Ade) synthetic dropout medium. The number at the top indicates three serial dilutions. AD, GAL4 activation domain; BD, GAL4 DNA-binding domain. b BiFC analysis of the interaction between Dt2 and GmAgl22. Scale bars, 10 mm. cYFP C-terminal portion of YFP. nYFP N-terminal portion of YFP. c Co-IP analysis of the protein interactions between Dt2 and GmAgl22. Flag-tagged GmAgl22 is co-transformed with HA-tagged Dt2 into Arabidopsis protoplasts. d Interaction between GmSoc1a and GmAgl22 in the yeast two-hybrid assay. e BiFC analysis of the interaction between GmSoc1a and GmAgl22. Scale bars, 10 mm. f Co-IP analysis of the protein interactions between GmSoc1a and GmAgl22. g Phenotypic comparison between W82 and GmSoc1a CR lines. Scale bars, 20 cm. h Branch number statistic in W82 and GmSoc1a CR lines ( n = 20 biologically independent plants). i Phenotypic comparison between DN50 and GmAgl22 OE lines. Scale bar, 10 cm. j Branch number statistic in DN50 and GmAgl22 OE lines ( n = 10 biologically independent plants). All the data in the graphs represent the mean ± SEM. Statistical significance is determined using a two-sided t -test. For ( b , e ), at least 5 independent cells are observed and a representative result is shown. For ( c , f ), at least 3 independent replicates are performed and a representative result is shown. Source data are provided as a Source Data file . Full size image Previously, we generated a GmSoc1a knockout mutant by the CRISPR/Cas9 system (named GmSoc1a CR ) and determined that the mutation could significantly affect flowering time. We also obtained two GmAgl22 overexpression lines (named GmAgl22 OE-1 and GmAgl22 OE-2 ) (Supplementary Fig. 10f ). We then compared the branch numbers of GmSoc1a CR and GmAgl22 OE with those of non-transgenic parents, respectively. We found that the GmSoc1a CR line showed significantly increased branch number (Fig. 3g, h ), and the GmAgl22 OE lines showed significantly decreased branch number (Fig. 3i, j ). These results indicated that Dt2, GmAgl22 and GmSoc1a may function by forming a complex to control branching in soybean. Dt2 regulates the expression of the GmAp1 gene family To mine the downstream targets and regulatory network of Dt2 , transcriptome profiling by RNA-Seq was performed with the lateral buds from WT (DN50), Dt2 CR and Dt2 OE . Using a P value < 0.05 and the fold change larger than 2 as thresholds, 646 up-regulated and 296 down-regulated genes were identified as differentially expressed genes (DEGs) between the wild type and Dt2 CR lines (WT/ Dt2 CR ) and 1160 up-regulated and 464 down-regulated genes were identified between the wild type and Dt2 OE lines (WT/ Dt2 OE ) (Supplementary Fig. 12a–d ). Gene Ontology (GO) term analysis demonstrated that the DEGs from the WT/ Dt2 CR and WT/Dt2 OE lines were enriched among metabolic process terms. Notably, multiple terms were related to carbohydrate metabolism and photosynthesis processes (Supplementary Fig. 12e, f ), which was consistent with previous findings that sugar metabolism or signaling played an important role in axillary bud outgrowth [1] , [25] , [26] . We then further narrowed down the DEGs by selecting the genes with an opposite pattern in the WT/ Dt2 OE and WT/ Dt2 CR panels: (1) up-regulated in the WT/ Dt2 OE panel but down-regulated in the WT/ Dt2 CR panel, and (2) down-regulated in the WT/ Dt2 OE panel but up-regulated in the WT/ Dt2 CR panel. In total, 30 genes meeting these criteria were identified (Fig. 4a ). Interestingly, half of these 30 genes were annotated as agamous-liked genes, and most of these agamous-liked genes showed higher expression in the shoot meristem and flower (Supplementary Fig. 13a ). Further comparison of the DEGs with previously reported Dt2 ChIP-seq data [20] revealed that 4 genes might be the direct targets of Dt2 : SoyZH13_16G083100 ( GmAp1a ), SoyZH13_01G060300 ( GmAp1c ), SoyZH13_02G112700 ( GmAp1d ) and SoyZH13_18G251400 ( GmRPP13 ). The three GmAp1 gene family members were significantly up-regulated in the Dt2 OE lines and down-regulated in the Dt2 CR line, whereas GmPRR13 was down-regulated in the Dt2 OE lines and up-regulated in the Dt2 CR lines (Fig. 4a and Supplementary Fig. 13b ). In this study, we focused on a functional assay of GmAp1 gene family using GmAp1a and GmAp1d as representatives. A previous in situ hybridization assay demonstrated that GmAp1a was specifically expressed in the shoot apices in the V2 stage [27] , and we also found that GmAp1a had a similar expression pattern as GmAp1d (Supplementary Fig. 13c ), indicating that they may perform a similar function in branching development. Fig. 4: Dt2 directly binds the promoter of GmAp1a and positively regulates its expression. a Venn diagram among overlapping DEGs from DN50, Dt2 CR and Dt2 OE lines. b A probe sequence that could be bound by the MADS-box protein in the promoter of the GmAp1a is predicted in Plantpan ( http://plantpan.itps.ncku.edu.tw/ ). c MBP-Dt2 HapI-1 or MBP-Dt2 HapI-2 directly bind to the promoter of GmAp1a in EMSA. MBP, maltose-binding protein. At least 3 independent replicates are performed and a representative result is shown. d , e Transient dual luciferase (dual-LUC) assays of Dt2 HapI-1 ( d ) and Dt2 HapI-2 ( e ) binding to the promoter of GmAp1a in tobacco leaves. f Transient dual luciferase (dual-LUC) assay of Dt2 on the promoter of GmAp1a in Arabidopsis protoplast ( n = 3 biologically independent replicates). Different letters indicate statistically significant differences at P < 0.05 by one-way ANOVA test. g , h Transient dual-LUC assay in tobacco leaves of Dt2 HapI-1 ( g ) or Dt2 HapI-2 ( h ) and its interacting proteins GmAgl22 and GmSoc1a on the promoter of GmAp1a . i Transient dual-LUC assay of Dt2 and its interacting proteins GmAgl22 and GmSoc1a on the promoter of GmAp1a in Arabidopsis protoplasts ( n = 3 biologically independent replicates). Different letters indicate statistically significant differences at P < 0.05 by one-way ANOVA test. j , k Phenotypic comparison between W82 and GmAp1a OE lines. Scale bars, 20 cm. l Branch number statistics of W82 and GmAp1a OE lines ( n = 20 biologically independent plants). Statistical significance is determined using a two-sided t -test. m , n Phenotypic comparison between the HX3 and GmAp1 4 m mutation lines in branch number. Scale bars, 20 cm. o Branch number statistics of the HX3 and GmAp1 4 m mutation lines ( n = 20 biologically independent plants). Data in ( f , i , l and o ) are mean ± SEM. Source data are provided as a Source Data file . Full size image A previous study showed that Dt2, a MADS-box protein, could bind to CArG elements [20] . Putative binding motif prediction using PlantPAN 3.0 ( http://plantpan.itps.ncku.edu.tw/ ) indicated that a sequence located −1274 bp from the GmAp1a translation initiation site (named Probe1) (Fig. 4b ) and a sequence located −678 bp from the GmAp1d translation initiation site (named Probe2) (Supplementary Fig. 14a ) might be the target sites of Dt2. Subsequently, we performed an electrophoretic mobility shift assay (EMSA) and found that the cold probe concentration could abolish the binding activities (Fig. 4c and Supplementary Fig. 14b ), confirming that Dt2 could bind to the promoters of GmAp1a and GmAp1d . Dt2-GmAgl22-GmSoc1a could activate the transcription of GmAp1a and GmAp1d To further explore how Dt2 affects the transcription of GmAp1 , we performed transient dual luciferase (Dural-LUC) assay in tobacco leaf system and Arabidopsis protoplasts. The results showed that Dt2 functioned as a transcriptional activator to promote the transcription of GmAp1a and GmAp1d (Fig. 4d–f and Supplementary Fig. 14c–e ), which was consistent with the changes in the expression of GmAp1 in Dt2 OE and Dt2 CR lines (Supplementary Fig. 13b ). Similarly, we found that Dt2-GmAgl22-GmSoc1a together showed stronger activity than Dt2 alone (Fig. 4g–i and Supplementary Fig. 14f–h ). To check whether GmAp1 indeed affects the branching of soybean, we overexpressed GmAp1a (named GmAp1a OE ) and also knocked out the four homologous genes of GmAp1 (named GmAp1 4m ) to eliminate their functional redundancy [27] . We found that the GmAp1a OE line exhibited significantly decreased branch number (Fig. 4j–l and Supplementary Fig. 13d ), and the quadruple mutant GmAp1 4m exhibited a significantly increased branch number (Fig. 4m–o and Supplementary Fig. 13e ), confirming that GmAp1 was indeed involved in branching development in soybean. Selection of Dt2 natural variations under adaptation Soybean is a vital crop in China and is planted nationwide from the high-latitude northeast to the low-latitude south. Since branching has a great influence on soybean yield, it has been considered and strongly selected in soybean breeding. Interestingly, we found that the branch number of the soybean accessions from different ecoregions exhibited significant differences: the average branch number of the accessions from higher latitudes was lower than that of accessions from lower latitudes (Fig. 5a ). Fig. 5: Geographic distribution of different Dt2 haplotypes and a proposed working model of Dt2 in controlling branch number in soybean. a Geographic distribution of Dt2 haplotypes in three different ecoregions. The column diagram is the percentage ratio between Dt2 HapI and Dt2 HapII . The bottom left box plot represents the branch number comparison of accessions in I ( n = 695 accessions), II ( n = 821 accessions) and III ( n = 222 accessions) ecoregions. Data are the mean ± SEM. In box plot (drawn by R 4.1.1 software), the center line indicates the median, the edges of the box represent the first and third quartiles, and the whiskers extend to span a 1.5 interquartile range from the edges. Different letters indicate statistically significant differences at P < 0.05 by one-way ANOVA test. b Proposed working model of the role of Dt2 in controlling branch number in soybean. IM inflorescence meristem. AM axillary meristem. SAM shoot apical meristem. The purple triangles represent the transitions from AM to IM. Full size image An investigation of the haplotypes of Dt2 using our 2898 previously re-sequenced accessions [15] revealed that Dt2 HapII did not exist in wild soybean and exhibited an increased ratio from landraces to cultivars (Supplementary Fig. 15a ). As Dt2 is a dominant locus controlling branching in soybean natural population (Fig. 1e, f ), we speculated that the natural variation in Dt2 may be related to the branch number variation in different planting ecoregions. We then investigated the haplotypes of Dt2 in the cultivated accessions (including landraces and cultivars) and found that the two Dt2 haplotypes exhibited different geographical distributions: an increased ratio of Dt2 HapI / Dt2 HapII from higher latitudes to the lower latitudes, which was consistent with the branch number change pattern (Fig. 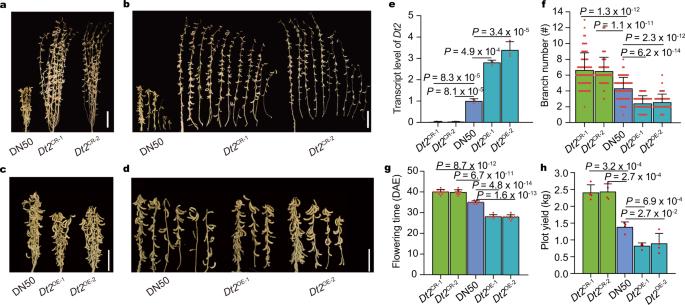Fig. 2: Dt2 negatively regulates the branch number. aArchitecture of DN50 andDt2CRplants at the harvest stage.bBranching ability of DN50 andDt2CRafter harvest.cArchitecture of DN50 andDt2OEplants at the harvest stage.dBranching ability of DN50 andDt2OEafter harvest.eRelative expression level ofDt2in DN50 and different transgenic lines (n= 3 biologically independent replicates).fBranch number of DN50,Dt2CRandDt2OElines (n= 70 biologically independent plants).gFlowering time of DN50,Dt2CRandDt2OElines (n= 30 biologically independent plants). DAE indicates days after emergence.hPlot yield of DN50,Dt2CRandDt2OE(n= 4 biologically independent replicates). The plot area is 10 m2. Scale bars in the (a–d) are 10 cm. Data in (e–h) are the mean ± SEM. Statistical significance is determined using a two-sidedt-test. Source data are provided as aSource Data file. 5a , Supplementary Table 2 and Supplementary Data 1 ). It has been suggested that the domestication of soybean may have originated in China in the Huanghuai region (ecoregion II in Fig. 5a ) and then radiated to the northern and southern regions [28] . F ST analysis showed that the Dt2 locus exhibited a genetic differentiation tendency between ecoregions II/I, but not between ecoregions II/III (Supplementary Fig. 15b ), indicating that the distinct geographic distribution of Dt2 haplotypes may be related to soybean adaptation to different latitudes. When a soybean accession from higher latitudes is planted at lower latitudes, it usually exhibits a significant yield decrease due to the early flowering and maturity [29] . The geographic and genetic differentiations of Dt2 inspired us that modification of Dt2 may improve the adaptation of soybean. DN50, the parent used for genetic modification of Dt2 in this study, is an accession from Heilongjiang Province (northeastern of China; 45°77′ N and 126°68′ E), a region located at high latitudes. 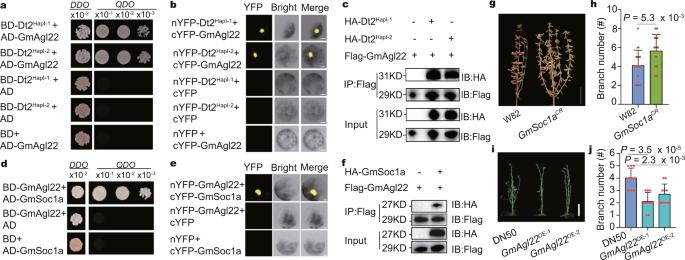Fig. 3: Dt2, GmAgl22 and GmSoc1a could interact with each other and affect the branch number. aInteraction between Dt2 and GmAgl22 in the yeast two-hybrid assay. Transformed yeast cells are grown onDDO(Trp/Leu) orQDO(Trp/Leu/His/Ade) synthetic dropout medium. The number at the top indicates three serial dilutions. AD, GAL4 activation domain; BD, GAL4 DNA-binding domain.bBiFC analysis of the interaction between Dt2 and GmAgl22. Scale bars, 10 mm. cYFP C-terminal portion of YFP. nYFP N-terminal portion of YFP.cCo-IP analysis of the protein interactions between Dt2 and GmAgl22. Flag-tagged GmAgl22 is co-transformed with HA-tagged Dt2 intoArabidopsisprotoplasts.dInteraction between GmSoc1a and GmAgl22 in the yeast two-hybrid assay.eBiFC analysis of the interaction between GmSoc1a and GmAgl22. Scale bars, 10 mm.fCo-IP analysis of the protein interactions between GmSoc1a and GmAgl22.gPhenotypic comparison between W82 andGmSoc1aCRlines. Scale bars, 20 cm.hBranch number statistic in W82 andGmSoc1aCRlines (n= 20 biologically independent plants).iPhenotypic comparison between DN50 andGmAgl22OElines. Scale bar, 10 cm.jBranch number statistic in DN50 andGmAgl22OElines (n= 10 biologically independent plants). All the data in the graphs represent the mean ± SEM. Statistical significance is determined using a two-sidedt-test. For (b,e), at least 5 independent cells are observed and a representative result is shown. For (c,f), at least 3 independent replicates are performed and a representative result is shown. Source data are provided as aSource Data file. When DN50 was planted in Beijing (in the middle of China; 40°22′ N and 116°23′ E) and Hainan (in the southern China, close to the equator; 18°09′ N and 108°48′E), the yields were significantly decreased (Supplementary Table 3 ). However, the Dt2 CR lines showed significantly higher yields than DN50, either at a lower planting density or a higher planting density, which was also associated with its effect on maturity (Supplementary Fig. 16 ). Shoot branching is both an agronomically important and a complex developmental trait that can be affected by many factors, of which the transition from the vegetative to reproductive stage is particularly important [30] , [31] . Functional variation in the genes related to vegetative-reproductive transition tends to cause a coupled phenotypic change in shoot branching morphology and flowering time, as observed, for the Hd3a gene in rice [32] and the VEG1 gene in pea [33] . In this study, we revealed that the dominant gene controlling branch number in soybean natural population, Dt2 , is a gene related to vegetative-reproductive transition. In addition, the interaction genes and downstream targets of Dt2 are also involved in flowering regulation [21] , [22] , [23] , [27] , [34] . Therefore, taking into account the abovementioned factors, we proposed a possible working model for the role of Dt2 in modulating soybean branching (Fig. 5b ): GmAp1 functions as a positive regulator in the transition from vegetative growth into reproductive growth by promoting the transition of axillary meristems (AM) into the inflorescence meristem (IM); Dt2 interacts with GmAgl22 and GmSoc1 to activate the transcription of GmAp1 ; the Dt2 HapII promoter has higher transcriptional activity than the Dt2 HapI promoter, which in turn enhances the expression of GmAp1 and promotes earlier transition from vegetative growth to reproductive growth, resulting in earlier flowering and reduced branching. Nevertheless, of the multiple polymorphisms between Dt2 HapI and Dt2 HapII , we have not disclosed the causal genetic variations responsible for the functional divergence of the two haplotypes. A further investigation of upstream regulatory genes may help us to determine which polymorphisms are essential for the transcription of Dt2 , which will make the regulatory network more complete. MADS-box transcription factor genes have been extensively studied in plants and were reported to play important roles in plant development, especially in vegetative-reproductive transition and plant architecture. 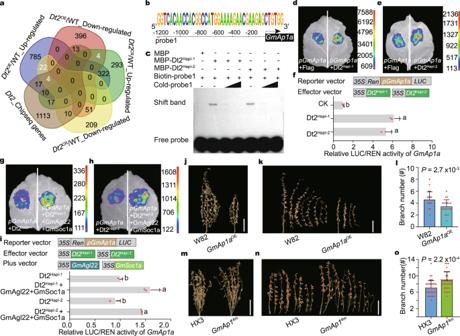Fig. 4: Dt2 directly binds the promoter of GmAp1a and positively regulates its expression. aVenn diagram among overlapping DEGs from DN50,Dt2CRandDt2OElines.bA probe sequence that could be bound by the MADS-box protein in the promoter of theGmAp1ais predicted in Plantpan (http://plantpan.itps.ncku.edu.tw/).cMBP-Dt2HapI-1or MBP-Dt2HapI-2directly bind to the promoter ofGmAp1ain EMSA. MBP, maltose-binding protein. At least 3 independent replicates are performed and a representative result is shown.d,eTransient dual luciferase (dual-LUC) assays of Dt2HapI-1(d) and Dt2HapI-2(e) binding to the promoter ofGmAp1ain tobacco leaves.fTransient dual luciferase (dual-LUC) assay of Dt2 on the promoter ofGmAp1ainArabidopsisprotoplast (n= 3 biologically independent replicates). Different letters indicate statistically significant differences atP< 0.05 by one-way ANOVA test.g,hTransient dual-LUC assay in tobacco leaves of Dt2HapI-1(g) or Dt2HapI-2(h) and its interacting proteins GmAgl22 and GmSoc1a on the promoter ofGmAp1a.iTransient dual-LUC assay of Dt2 and its interacting proteins GmAgl22 and GmSoc1a on the promoter ofGmAp1ainArabidopsisprotoplasts (n= 3 biologically independent replicates). Different letters indicate statistically significant differences atP< 0.05 by one-way ANOVA test.j,kPhenotypic comparison between W82 andGmAp1aOElines. Scale bars, 20 cm.lBranch number statistics of W82 andGmAp1aOElines (n= 20 biologically independent plants). Statistical significance is determined using a two-sidedt-test.m,nPhenotypic comparison between the HX3 andGmAp14mmutation lines in branch number. Scale bars, 20 cm.oBranch number statistics of the HX3 andGmAp14mmutation lines (n= 20 biologically independent plants). Data in (f,i,lando) are mean ± SEM. Source data are provided as aSource Data file. 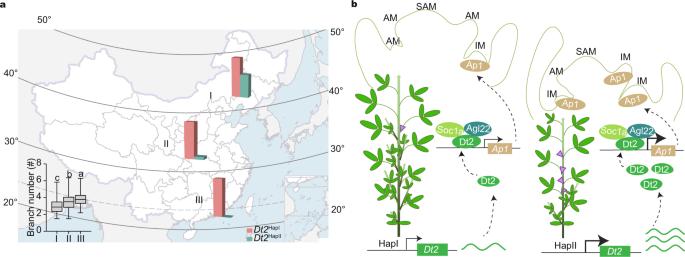Fig. 5: Geographic distribution of different Dt2 haplotypes and a proposed working model of Dt2 in controlling branch number in soybean. aGeographic distribution ofDt2haplotypes in three different ecoregions. The column diagram is the percentage ratio betweenDt2HapIandDt2HapII. The bottom left box plot represents the branch number comparison of accessions in I (n= 695 accessions), II (n= 821 accessions) and III (n= 222 accessions) ecoregions. Data are the mean ± SEM. In box plot (drawn by R 4.1.1 software), the center line indicates the median, the edges of the box represent the first and third quartiles, and the whiskers extend to span a 1.5 interquartile range from the edges. Different letters indicate statistically significant differences atP< 0.05 by one-way ANOVA test.bProposed working model of the role ofDt2in controlling branch number in soybean. IM inflorescence meristem. AM axillary meristem. SAM shoot apical meristem. The purple triangles represent the transitions from AM to IM. For instance, SUPPRESSOR OF OVEREXPRESSION OF CO1 and FRUITFULL were found to not only promote flowering, but also affect the determinacy of meristems in Arabidopsis [35] . Previous studies in soybean have illuminated that the members involved in the working model of Dt2 from this study, including Dt2 , GmAgl22 , GmSoc1 and GmAp1 , all regulate flowering time by being involved in inflorescence transition [18] , [19] , [20] , [24] , [27] . Similarly, MtFUL1-c and VEG1 / PsFUL1-c , orthologs of Dt2 from Medicago and pea respectively, were also found to play important roles in the reproductive phase transition [33] , [36] . Here, we found that these genes not only affect flowering time, but also control branch number in soybean. Consistently, the Arabidopsis homologs of Dt2 - GmSoc1a , FUL - SOC1 , were also found to regulate branch number [35] , [37] , [38] . These results suggested that Dt2 and other MADS box genes are highly pleiotropic in regulating vegetative-reproductive transition and plant architecture. In addition, these results also indicated that the network of MADS box genes in regulating plant architecture may be functionally conserved among plant species. Taken together previous studies [18] , [19] , [20] , [24] , [27] , our results revealed that Dt2, GmAgl22 and GmSoc1 function as a complex to regulate GmAp1 . Interestingly, the genes involved in the working model of Dt2 all belong to the MADS-box gene family, indicating a complicated regulatory network among different MADS-box transcription factor genes although they belong to the same transcription factor family. Further investigation of more MADS-box members is needed to reveal more detailed regulatory networks of this important transcription factor gene family. Soybean was originally domesticated in China and was then introduced into different countries [39] . Because soybean is highly sensitive to photoperiod, selection of the beneficial alleles of the genes that confer adaptation is critical during the spreading process [13] , [40] . For instance, selection of natural variation in the J gene improved the soybean adaptation to the tropical regions and significantly enhanced yield [29] , making Brazil one of the largest soybean producing countries today. Here, we determined that the natural variation in Dt2 is also related to the adaptation of soybean (Fig. 5a , Supplementary Fig. 15 ), which provides a genetic candidate for adaptation breeding in soybean. In the future, a trial involving a combinational selection/modification of J and Dt2 may enhance soybean adaptation ability. In addition to the vegetative-reproductive transition, other factors/pathways also determine shoot branching development [1] . Here, we found that the dominant gene associated with branch number in soybean is related to vegetative-reproductive transition. Next, fixing the effect of vegetative-reproductive transition, particularly the effect of the dominant gene Dt2 may help to identify additional genes functioning in sobyean shoot branching, and will provide more insight for soybean improvement. Plant materials and growth conditions The 2409 soybean accessions used for the GWAS were planted at the experimental station of the Tianjin Academy of Agricultural Science, Wuqing (39° 38′ N and 117° 04′ E) during the summer season in 2017 and the Institute of Genetics and Developmental Biology, Chinese Academy of Sciences, Beijing (40° 22′ N and 116° 23′ E) in 2018. At the full-pod stage (R4), 5 representative plants were selected from each accession and the primary effective branch number was identified. The Dt2 HapI-1 material was PI 548533 and Dt2 HapII was PI 547501. For the BiFC and dual Luciferase reporter assays, Arabidopsis ecotype Col-0 was planted in the greenhouse at 22 °C under an 8 h light and 16 h dark photoperiod. Tobacco ( Nicotiana benthamiana ) was planted in the greenhouse at 22 °C under a 16 h light and 8 h dark photoperiod. Vector construction and transformation To construct the Dt2 overexpression plasmid, the CDS of Dt2 was amplified from DN50 and ligated into pTF101, a binary vector containing the CaMV 35 S promoter and a terminator, with the restriction sites XbaI and SacI. To construct the GmAgl22 overexpression plasmid, the CDS of GmAgl22 was ligated into pTF101 with the restriction sites XbaI and SacI. These constructs were introduced into Agrobacterium tumefaciens strain EHA101 and then transformed into DN50. For the CRISPR/Cas9 system experiments, two sgRNAs were designed using Primer Design software. Two U6 promoters were used for the guide RNA oligonucleotide pair. The U6 promoter driving a single guide RNA cassette was cloned into the PMDC123 vector [41] . These constructs were introduced into Agrobacterium tumefaciens strain EHA105 and then transformed into DN50. The relevant primers used are listed in Supplementary Data 2 . RNA extraction and expression analysis Total RNA was extracted using an RNA isolation kit (Tiangen, DP432) according to the manufacturer’s protocol and three biological replicates were performed in each experiment. Reverse transcription was performed using a cDNA synthesis kit (Transgen, AE311). Then the cDNA sequence was used as the template for the quantitative real-time PCR. qPCR was performed using LightCycler 480 SYBR Green I Master (Transgen, AQ101-01) on a LightCycler 480 instrument (Roche). Gene expression was normalized to the expression of the soybean gene ACTIN11 . Fold changes were calculated from the 2 −ΔΔCt values. The relevant primers used are listed in Supplementary Data 2 . GWAS analysis For GWAS, we used the previously reported SNP dataset [15] . A total of 4,072,231 SNPs were used for association analysis with a minor allele frequency (MAF) of >5% and a missing rate of <10%. GWAS was performed based on a mixed model using the EMMAX software package [42] . EIGENSOFT software [43] was used to perform principal-component analysis of the population, and the first five principal components were included as fixed effects. The matrix of pairwise genetic distances derived from the simple matching coefficients was used as the variance-covariance matrix of the random effects. For the threshold, we defined the whole-genome significance cutoff as the Bonferroni test threshold [44] , [45] , the threshold was set as −log(0.05/total SNPs), and the genome-wide significance level for branch number was determined as 1 × 10 −7.9 . Haplotype analysis of Dt2 in the soybean population The SNPs in the 3.5 kb promoter region and full-length genomic region of Dt2 of 2409 varieties were obtained from the previously reported SNP and INDEL dataset [15] . Then the SNPs were filtered by applying a MAF > 5% cutoff, missing rate <10%, nonfunctional SNP mutation and low association signals SNPs, retaining 35 high-quality SNPs. The association polymorphisms classified the accessions into three major haplotypes. Phylogenetic tree analysis The homology of Dt2 proteins was searched in Phytozome 13 ( https://phytozome-next.jgi.doe.gov/blast-search ), focusing on genes with homology >50% in soybean, Arabidopsis and rice. MEGA 6.0 was used for sequence comparison and phylogenetic tree construction analysis and the bootstrap repetition value was 1000. The phylogenetic tree was further modified by the online tool evolview ( https://www.evolgenius.info//evolview/ ) [46] . Selection analysis The genetic differentiation fixation index ( F ST ) was calculated by using VCFtools (0.1.13) with a 20 kb slide window and 2 kb slide step [47] . The first 5% value was used as the threshold in the whole genome. In situ hybridization In situ hybridization treatments were performed as previously described [48] , [49] . Briefly, the soybean shoot apexes of 10, 16 and 22 day-old seedlings were fixed in 50% formol-acetic-alcohol. Subsequently, the 8 μm-thick SAM samples slices were observed in a conventional light microscope after sample fixation, embedding, sectioning and hybridization. The size of the Dt2 probe was 228 bp, that of the GmAgl22 probe was 137 bp, and that of the GmSoc1a probe was 140 bp. The primers are listed in Supplementary Data 2 . RNA-seq sample preparation and sequencing Lateral buds from the same node of WT and transgenic soybean plants were collected for RNA-seq analysis. Three biological replicates were performed for each sample. The Illumina HiSeq 2000 platform was used to generate 150 bp paired-end reads. And the detailed bioinformatic analyses were performed as previously described [50] . Briefly, the high-quality sequencing reads were mapped to the reference genome with Hisat (v. 2.2.1). And the gene expression counts were calculated using StringTie (v.1.3.4d). The different expression genes analysis were analyzed by the R-edgeR library ( https://bioconductor.org/packages/release/bioc/html/edgeR.html ). Yeast two-hybrid assays Yeast two-hybrid assays were performed as described in the Yeast Protocols Handbook (Clontech). The coding region sequence of Dt2 HapI-2 was introduced into the prey vector (pGBKT7). To construct the prey vectors, we ligated the full-length CDSs of GmAgl22 and GmSoc1a into the pGADT7 vector. Then pGBKT7- Dt2 HapI-2 was transformed into the Y2HGold strain with pGADT7- GmAgl22 or pGADT7- GmSoc1a and selected on DDO (Synthetic Dropout Medium/-Tryptophan-Leucine) and QDO (Synthetic Dropout Medium/-Tryptophan-Histone-Leucine-Adenine) media (Clontech). The empty AD or empty BD served as a negative control. The primers are listed in Supplementary Data 2 . BiFC For the construction of BiFC vectors, the Gateway-compatible vectors pUGW2-nYFP and pUGW2-cYFP were used to generate vectors in BIFC assays by using Gateway cloning technology. pUGW2-nYFP is the vector for N-terminal fusion to yellow fluorescent protein (nYFP), and pUGW2-cYFP is the vector for C-terminal fusion to YFP (cYFP). The full-length CDS of Dt2 HapI-2 was cloned into pUGW2-nYFP. The full-length CDSs of GmAgl22 and GmSoc1a were cloned into pUGW2-cYFP. Arabidopsis protoplasts were prepared for the expression assays. Vectors were co-transformed into Arabidopsis protoplasts and incubated at 22 °C in the dark for 12–16 h. YFP fluorescence was visualized using confocal laser scanning microscope (Zeiss LSM 985 NLO). Co-IP analysis Co-IP analysis was performed using Arabidopsis protoplasts [47] . To construct the vector, full-length CDSs of Dt2 HapI-1 and Dt2 HapI-2 were cloned into pUC19- 35S -HA vectors, and the CDSs of GmAgl22 and GmSoc1a were introduced into the pUC19- 35S -Flag vector. A. thaliana protoplasts were transfected with 50 μg of plasmid and incubated overnight under low-light-intensity environment. Total protein was extracted from protoplasts after incubation for 12–16 h using extraction buffer (50 mM Tris-HCl (pH 7.5), 0.5 mM EDTA, 150 mM NaCl, 0.5% np-40, 1 mM PMSF, and 1× complete protease inhibitor cocktail (Roche, 04693132001). The protein lysis product were incubated with Flag magnetic beads (MBL) for 30 min to 1 h and wash the beads four times with a wash buffer that consisted of 50 mM Tris-HCl (pH 7.5), 150 mM NaCl, 20% glycerol, 0.1% Triton X-100, 1 mM EDTA (pH 8.0) and 1× complete protease inhibitor cocktail. The immunoprecipitates were separated using SDS-PAGE and transferred to a nitrocellulose membrane (GE Healthcare). Proteins were detected by treating the membranes with anti-HA (1:5,000, MBL, M180-7) or anti-DDDDK-tag mAb-HRP-DirectT antibodies (1:10,000, MBL, M185-7). Transient dual luciferase (dual-LUC) assay To generate the pGmAp1a :LUC and pGmAp1d :LUC constructs, we amplified 3-Kb promoter fragments upstream of each gene from Williams 82 and ligated them with the pGreen0800-LUC as the reporter vector. The p35S - Dt2 HapI-1 -Flag, p35S - Dt2 HapI-2 -Flag, p35S - GmAgl22 -Flag and p35S - GmSoc1a -Flag constructs were used as effectors. Transient transactivation assays were performed using Arabidopsis protoplasts [51] . In the tobacco leaf system, the promoters of the GmAp1a and GmAp1d (3000 bp) were cloned into the transient expression vector CP461, which was constructed as the reporter vector. In addition, the p35S - Dt2 HapI-1 -Flag, p35S - Dt2 HapI-2 -Flag, p35S - GmAgl22 -Flag and p35S - GmSoc1a -Flag constructs were used as effectors and these plasmids were transformed into A. tumefaciens strain GV3101. Then these strains were injected into tobacco leaves in different combinations with p19, which was used to suppress RNA silencing. Dual luciferase assay reagents (Promega, VPE1910) with the Renilla luciferase gene as an internal control were used for luciferase imaging. The relevant primers are listed in Supplementary Data 2 . Split luciferase (split-LUC) complementation assay Luciferase complementation imaging assays were performed as described previously [52] . Briefly, to generate a luciferase complementation vector, pCAMBIA1300- 35S -NLuc was fused with the C- termini of Dt2 HapI-1 , Dt2 HapI-2 and GmAgl22 , and pCAMBIA1300- 35S -CLuc was fused with the C-termini of GmAgl22 and GmSoc1a . Transient expression in tobacco ( Nicotiana benthamiana ) leaves was conducted by GV3101 Agrobacterium infiltration. Plants were then incubated at 22 °C for 2 days before the LUC activity was measured. Images were captured using the low-light cooled charge-coupled device imaging apparatus NightOWL IILB 983. Electrophoretic mobility shift assay The full length of Dt2 HapI-1 and Dt2 HapI-2 CDSs were amplified and cloned into the Pmal-C5x vector. MBP-Dt2 HapI-1 and MBP-Dt2 HapI-2 recombinant proteins with MBP tags were introduced into Escherichia coli BL21 (DE3). The recombinant proteins were purified by using maltose resin (NEB, E8021S). DNA probes (Probe1 in GmAp1a and Probe2 in GmAp1d ) were artificially synthesized and labeled with biotin at the 5′ end (Thermo Fisher Scientific). DNA gel shift assays were performed as the protocol described of the LightShift Chemiluminescent EMSA kit (Thermo Fisher Scientific, 20148). The probe sequences are listed in Supplementary Data 2 . Reporting summary Further information on research design is available in the Nature Research Reporting Summary linked to this article.